Correspondence: Quantitative evaluation of X-ray dark-field images for microcalcification analysis in mammography 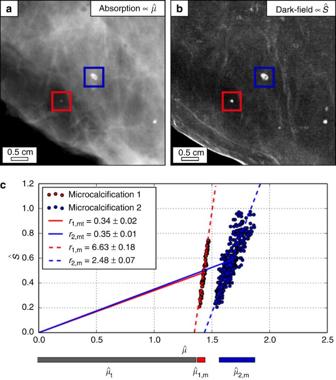Figure 1: Quantitative evaluation of microcalcification analysis in X-ray dark-field mammography. (a) Experimental absorption and (b) dark-field mammogram of a freshly dissected breast abladate with microcalcifications. (c) Scatter plots comparing the absorptionto scattering powerof two exemplary microcalcifications cluster, as indicated by the blue and red frame in (a,b), respectively. An incorrectr-value is obtained (rWang=rmt) if contributions of the underlying tissue are neglected in the analysis, since>>. How to cite this article: Scherer, K. et al. Correspondence: Quantitative evaluation of X-ray dark-field images for microcalcification analysis in mammography. Nat. Commun. 7:10863 doi: 10.1038/ncomms10863 (2016).